Spatial control of Cdc42 signalling by a GM130–RasGRF complex regulates polarity and tumorigenesis The small GTPase Cdc42 is a key regulator of polarity, but little is known in mammals about its spatial regulation and the relevance of spatial Cdc42 pools for polarity. Here we report the identification of a GM130–RasGRF complex as a regulator of Cdc42 at the Golgi. Silencing GM130 results in RasGRF-dependent inhibition of the Golgi pool of Cdc42, but does not affect Cdc42 at the cell surface. Furthermore, active Cdc42 at the Golgi is important to sustain asymmetric front–rear Cdc42-GTP distribution in directionally migrating cells. Concurrent to Cdc42 inhibition, silencing GM130 also results in RasGRF-dependent Ras-ERK pathway activation. Moreover, depletion of GM130 is sufficient to induce E-cadherin downregulation, indicative of a loss in cell polarity and epithelial identity. Accordingly, GM130 expression is frequently lost in colorectal and breast cancer patients. These findings establish a previously unrecognized role for a GM130–RasGRF–Cdc42 connection in regulating polarity and tumorigenesis. Cell polarity is a highly orchestrated multi-step cellular process that regulates a plethora of biological functions of relevance for cell migration, wound healing and cancer. Among the regulators of polarity, the small GTPase Cdc42 plays a central role [1] . Given the emerging role of polarity in tumorigenesis [2] , [3] , [4] , it is now important to study the regulation of Cdc42 in time and space. A large body of evidence exists on Cdc42 signalling at or from the plasma membrane, but comparatively little is known about Cdc42 signalling from endomembranes such as the Golgi apparatus, where this Rho family GTPase has been detected previously [5] , [6] . It currently remains unclear whether Cdc42 at the Golgi is regulated, what factors contribute to its activation and whether this pool is of any relevance for cell polarity. Endomembranes are increasingly recognized as sites where cellular signals are either initiated or modulated [7] , thus supporting the notion that the Golgi pool of Cdc42 might be biologically relevant. Furthermore, the Golgi apparatus is known to play a role in directional migration and polarity [8] , but there is surprisingly little mechanistic understanding of the role of this organelle in directional motility and cell polarity. Therefore, investigating whether a Golgi protein regulates spatial Cdc42 signalling might provide mechanistic insight into the role of the Golgi in polarity. RasGRF family Guanine Nucleotide Exchange Factors (GEFs) are well-known regulators of the small GTPase Ras [9] , [10] . In addition, RasGRFs mediate functional crosstalk between Ras signalling and Cdc42 (refs 11 , 12 ). In this respect, it has been recently demonstrated that RasGRF binds to and inhibits Cdc42, thereby regulating cellular motility, transformation and invasion [13] . In the current work, we find that the Golgi matrix protein GM130 might regulate the activity of the Golgi pool of Cdc42. Through short interfering RNA (siRNA) screening of a GEF library, we identified candidate GEFs that contribute to the regulation of Cdc42 specifically at the Golgi, but surprisingly none of these is involved in regulating the GM130–Cdc42 axis. We then identified RasGRF2 as a novel interaction partner for GM130 and demonstrate that this interaction is pivotal for the regulation of both Ras and Cdc42. Loss of GM130 releases RasGRF, allowing it to inhibit Cdc42 and activate Ras, leading to alterations in cell polarity and hyperactivity of the Ras-ERK pathway. Importantly, we show that GM130 is frequently downregulated in cancer. The Golgi pool of Cdc42 controls cell polarity To study spatial Cdc42 activation patterns we used a Cdc42 Raichu probe [14] , [15] . For all our measurements we used a probe containing the C-terminal domain of Cdc42 (ref. 15 ) (Cdc42-EM hereafter). This C-terminal domain targets the Fluorescence Resonance Energy Transfer (FRET) reporter to different membranes including the plasma membrane and various cellular endomembranes such as the Golgi and endosomes ( Supplementary Fig. 1A ), localizing as reported for endogenous Cdc42 (ref. 5 ). Cdc42-EM appeared in a juxtanuclear pool colocalizing with GM130, indicating its presence at the Golgi complex ( Supplementary Fig. 1B ), thus allowing us to monitor Cdc42 activation at this cellular location [6] ( Fig. 1a ). Measuring FRET outside the Golgi area or the plasma membrane did not reveal any specific signal, thus supporting the specificity of our FRET measurements ( Fig. 1a ). Silencing GM130 reduced the total cellular pool of Cdc42-GTP (ref. 16 ) ( Supplementary Fig. 1C ), and specifically reduced the activity of Cdc42 at the Golgi ( Fig. 1b ). However, GM130 depletion did not affect the activity of the reporter at the plasma membrane ( Fig. 1c ). Silencing GM130 inhibited two-dimensional (2D) cell migration ( Supplementary Fig. 1E ), indicating that alteration of spatial Cdc42 signalling is relevant for directed cell motility. Moreover, the recruitment of aPKC to the leading edge of directionally migrating cells was also reduced ( Supplementary Fig. 1F ). To test for effects on polarity in a 3D cell culture model, we used Caco-2 cells, which are known to spontaneously polarize when plated in a 3D matrix, forming cysts with a single lumen. Previous work showed that alteration of Cdc42 activity leads to the formation of multi-lumen (aberrant) cysts [17] , [18] . Depletion of GM130 in Caco-2 cells led to an increase in the number of aberrant cysts, which is indicative of a polarity defect ( Fig. 1d ). These results suggested that regulation of spatial Cdc42 activity by GM130 was relevant for cell polarization in 2D and 3D cell culture. In contrast, GM130 depletion did not affect Golgi morphology ( Supplementary Fig. 2 ), endoplasmic reticulum (ER)–Golgi trafficking, Golgi-to-plasma membrane trafficking or coatomer recruitment to the Golgi ( Supplementary Fig. 3A–C ). Furthermore, the capability of the Golgi to nucleate microtubules was also unaffected ( Supplementary Fig. 3D ), in agreement with previous findings [19] . Thus, the indirect impact of these processes on polarity could be excluded [8] . 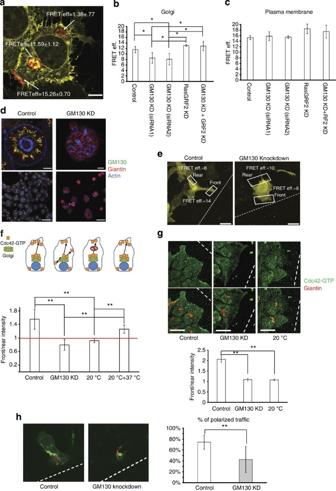Figure 1: GM130 spatially regulates Cdc42 activity to control polarity. (a) Representative HEK293 cell expressing the Cdc42-EM-FRET reporter. Areas where FRET was measured are marked in red and average FRET values±s.d. are shown. Scale bar, 25 μm. (b,c) FRET-based measurement of Cdc42 activity at the Golgi (b) or plasma membrane (c). Averages of three experiments±s.d. (minimum 15 cells per condition per experiment) are shown. (d) Caco-2 cells were transfected with the indicated siRNA were grown in Geltrex for 4 days and cysts were stained for Giantin (red) and GM130 (green) and with phalloidin (blue). Scale bars, 7.5 μm and 75 μm for the upper and lower image, respectively. (e,f) HeLa cells expressing the Cdc42-EM probe were transfected with the indicated siRNA. A wound was introduced and cells were allowed to polarize for 6 h. FRET was measured on the plasma membrane part facing the wound (Front) and on the opposing end of the cell (Rear). Scale bar, 10 μm. Bar graph represents FRET measurements from three independent experiments. Above, the graph schematics of the experimental setup are displayed. Results are presented as mean±s.d. from four experiments. White lines indicate position of the wound. 20 °C: cells incubated at 20 °C for 2 h before FRET measurement. 20+37 °C: cells incubated at 20 °C for 2 h before followed by rewarming at 37 °C. (g) Same experimental setup as ine,fexcept no FRET reporter was used, but Cdc42-GTP was immunostained. Cdc42-GTP intensities were measured and the front/rear ratio is plotted as a bar graph. Results are presented as mean±s.d. of three experiments. Scale bar, 25 μm. (h) Confluent monolayer of HeLa cells expressing VSVG-RUSH–GFP was wounded and cells were allowed to migrate for 6 h followed by addition of biotin to release VSVG from the ER. 25 min after biotin addition, carriers were imaged by live video microscopy. Individual tracks measured by ImageJ are displayed on the representative images. Results are presented as mean±s.d. from three experiments. Statistics ina–g: analysis of variance with Newman–Keuls multiple comparison test (*P<0.05; **P<0.01). Inh: Student’st-test (**P<0.01). Figure 1: GM130 spatially regulates Cdc42 activity to control polarity. ( a ) Representative HEK293 cell expressing the Cdc42-EM-FRET reporter. Areas where FRET was measured are marked in red and average FRET values±s.d. are shown. Scale bar, 25 μm. ( b , c ) FRET-based measurement of Cdc42 activity at the Golgi ( b ) or plasma membrane ( c ). Averages of three experiments±s.d. (minimum 15 cells per condition per experiment) are shown. ( d ) Caco-2 cells were transfected with the indicated siRNA were grown in Geltrex for 4 days and cysts were stained for Giantin (red) and GM130 (green) and with phalloidin (blue). Scale bars, 7.5 μm and 75 μm for the upper and lower image, respectively. ( e , f ) HeLa cells expressing the Cdc42-EM probe were transfected with the indicated siRNA. A wound was introduced and cells were allowed to polarize for 6 h. FRET was measured on the plasma membrane part facing the wound (Front) and on the opposing end of the cell (Rear). Scale bar, 10 μm. Bar graph represents FRET measurements from three independent experiments. Above, the graph schematics of the experimental setup are displayed. Results are presented as mean±s.d. from four experiments. White lines indicate position of the wound. 20 °C: cells incubated at 20 °C for 2 h before FRET measurement. 20+37 °C: cells incubated at 20 °C for 2 h before followed by rewarming at 37 °C. ( g ) Same experimental setup as in e , f except no FRET reporter was used, but Cdc42-GTP was immunostained. Cdc42-GTP intensities were measured and the front/rear ratio is plotted as a bar graph. Results are presented as mean±s.d. of three experiments. Scale bar, 25 μm. ( h ) Confluent monolayer of HeLa cells expressing VSVG-RUSH–GFP was wounded and cells were allowed to migrate for 6 h followed by addition of biotin to release VSVG from the ER. 25 min after biotin addition, carriers were imaged by live video microscopy. Individual tracks measured by ImageJ are displayed on the representative images. Results are presented as mean±s.d. from three experiments. Statistics in a – g : analysis of variance with Newman–Keuls multiple comparison test (* P <0.05; ** P <0.01). In h : Student’s t -test (** P <0.01). Full size image Directed trafficking causes asymmetric distribution of Cdc42 To obtain direct evidence for the role of the GM130-regulated Golgi pool of active Cdc42, we measured Cdc42 activity at the front and the rear of directionally migrating cells using the Cdc42-EM probe. Strikingly, Cdc42 activity exhibited an asymmetric distribution, being more active at the front compared with the rear of the cell ( Fig. 1e,f ). Silencing GM130 reduced the amount of activated Cdc42 at the leading edge, thereby breaking the asymmetric distribution of active Cdc42 ( Fig. 1e,f ). These results were confirmed by immunofluorescence staining of endogenous Cdc42-GTP ( Fig. 1g ). Sustained accumulation of active Cdc42 at the leading edge could be the consequence of an increased local activation. Alternatively, the Golgi might deliver Cdc42-GTP to the leading edge. If the latter mechanism is true, then blocking trafficking from the Golgi ought to diminish the amount of Cdc42-GTP at the leading edge. To test this point, directionally migrating cells in a wound closure assay were incubated at 20 °C for 1 h, which blocks exit from the trans-Golgi [20] . Measuring FRET reporter activity or staining for Cdc42-GTP revealed that blocking post-Golgi trafficking diminished the presence of GTP-Cdc42 at the cell front, thereby abolishing Cdc42-GTP asymmetry ( Fig. 1e,f ). Importantly, re-incubation of the cells at 37 °C for 1 h re-established Cdc42-GTP asymmetry with higher levels at the leading edge compared with the rear ( Fig. 1f ). The loss of Cdc42-GTP asymmetry in GM130 knockdown cells was likely due to abrogation of directed trafficking. Live cell imaging of green fluorescent protein (GFP)–VSVG tracks forming from the Golgi showed that while carriers formed readily in GM130-depleted cells, they were non-directed, contrary to tracks in control cells, which mostly trafficked towards the leading edge ( Fig. 1h ). Of note, the directionality of post-Golgi trafficking was affected, whereas the global rate of post-Golgi trafficking was not ( Supplementary Fig. 3B ). Since, both GDP- and GTP-restricted Cdc42 is known to block post-Golgi trafficking [21] we conclude that GM130 depletion does not affect the GTP/GDP cycling of Cdc42. Taken together, the Golgi pool of active Cdc42 is relevant for cell polarization. The GM130–Cdc42 crosstalk does not involve GEFs Next we asked how the Cdc42 activity at the Golgi is regulated by GM130. One possibility is that GM130 recruits a Cdc42–GEF leading to local activation of this GTPase. If true, then this GEF must interact with GM130 and localize to the Golgi in a GM130-dependent manner (schematic in Fig. 2 ). 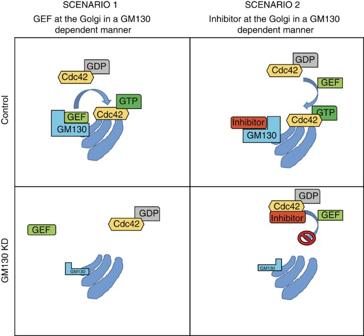Figure 2: Models for the GM130–Cdc42 crosstalk. Schematic representation of two different models. On the left-hand side: GM130 acts as a scaffold for a Cdc42–GEF at the Golgi. In this case, a GEF should be located at the Golgi in a GM130-dependent manner. Upon GM130 depletion, the GEF is lost from the Golgi and subsequently, Cdc42-GTP doesn’t accumulate at the organelle. In the second scenario (right-hand side), GM130 binds to an inhibitor of Cdc42, protecting the small GTPase from inactivation. If GM130 is lost, the inhibitor will bind to Cdc42 in places other than the Golgi, thereby preventing a GEF-mediated activation of Cdc42. In this way, Cdc42-GTP will not be accumulated at the Golgi. Figure 2: Models for the GM130–Cdc42 crosstalk. Schematic representation of two different models. On the left-hand side: GM130 acts as a scaffold for a Cdc42–GEF at the Golgi. In this case, a GEF should be located at the Golgi in a GM130-dependent manner. Upon GM130 depletion, the GEF is lost from the Golgi and subsequently, Cdc42-GTP doesn’t accumulate at the organelle. In the second scenario (right-hand side), GM130 binds to an inhibitor of Cdc42, protecting the small GTPase from inactivation. If GM130 is lost, the inhibitor will bind to Cdc42 in places other than the Golgi, thereby preventing a GEF-mediated activation of Cdc42. In this way, Cdc42-GTP will not be accumulated at the Golgi. Full size image To identify GEFs that contribute to activate Cdc42 at the Golgi, we screened a library of 51 siRNAs against Rho family GEFs for effects on the Golgi pool of Cdc42 using the Cdc42-EM-FRET probe. We focused primarily on the knockdowns that affected Cdc42 activity at the Golgi more strongly than GM130 depletion. While several GEF knockdowns decreased the FRET values at the Golgi, only three had an effect that was comparable to the effect of GM130, namely ARHGEF9, 11 and 12 ( Fig. 3a ). Depletion of GEF11 and 12 also resulted in reduced total cellular Cdc42-GTP ( Supplementary Fig. 4B ), supporting these FRET measurements. Depletion of any of these GEFs also resulted in an inhibition of directed migration as determined in a wound-healing assay ( Supplementary Fig. 4C ). In addition, polarization of the Golgi to the leading edge of migrating cells was also affected ( Supplementary Fig. 4D ). However, none of these GEFs interacted with GM130 in co-immunoprecipitation experiments, nor did they localize to the Golgi ( Fig. 3b,c ). We also failed to detect any evidence for an involvement of the GEF Tuba, as it did not localize to the Golgi ( Supplementary Fig. 5A,B ), nor did it interact with GM130 ( Supplementary Fig. 5C,D ) contrarily to previous findings [16] , and in agreement with others who failed to detect this GEF at the Golgi [22] , [23] . In addition, neither Tuba depletion ( Fig. 3a , Supplementary Fig. 5E ) nor its overexpression ( Supplementary Fig. 5F ) changed the activation of Cdc42 at the Golgi. Of note, none of the GEFs tested localizes to the Golgi (Oliver Rocks, personal communication). Therefore, the GM130–Cdc42 crosstalk is not mediated via recruitment of a GEF driving local activation of Cdc42. 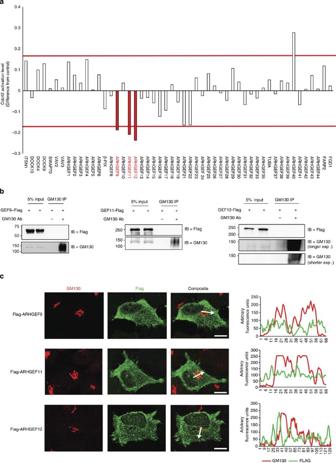Figure 3: Screening for GEFs that regulate the Golgi pool of Cdc42. (a) HEK293 cells were transfected with control or with the indicated siRNA. After 48 h, cells were transfected with the plasmid encoding for the Cdc42-EM-FRET probe. After a further 24 h the cells were fixed and mounted. FRET was measured as described in the Methods section and FRET values are displayed as fold of control and are averages from the measurements of at least 30 cells per condition. Red bars represent CI95 intervals (b) HeLa cells were transfected with plasmids encoding the indicated GEF. Twenty-four hours later, cells were lysed and the lysates were subjected to immunoprecipitation either with a GM130 antibody (+) or with protein G sepharose beads alone. ‘5% input’ indicates lanes where 5% of the total material that was used in the immunoprecipitation is loaded. The immunoprecipitated material was eluted and subjected to SDS–polyacrylamide gel electrophoresis followed by immunoblotting against the indicated proteins. (c) HeLa cells were plated on coverslips, then transfected with plasmids encoding the specified GEF. Twenty-four hours later, cells were fixed and immunostained for GM130 and Flag. Intensity plot corresponding to the region marked by a white arrow are shown on the right. Scale bar, 10 μm. Figure 3: Screening for GEFs that regulate the Golgi pool of Cdc42. ( a ) HEK293 cells were transfected with control or with the indicated siRNA. After 48 h, cells were transfected with the plasmid encoding for the Cdc42-EM-FRET probe. After a further 24 h the cells were fixed and mounted. FRET was measured as described in the Methods section and FRET values are displayed as fold of control and are averages from the measurements of at least 30 cells per condition. Red bars represent CI95 intervals ( b ) HeLa cells were transfected with plasmids encoding the indicated GEF. Twenty-four hours later, cells were lysed and the lysates were subjected to immunoprecipitation either with a GM130 antibody (+) or with protein G sepharose beads alone. ‘5% input’ indicates lanes where 5% of the total material that was used in the immunoprecipitation is loaded. The immunoprecipitated material was eluted and subjected to SDS–polyacrylamide gel electrophoresis followed by immunoblotting against the indicated proteins. ( c ) HeLa cells were plated on coverslips, then transfected with plasmids encoding the specified GEF. Twenty-four hours later, cells were fixed and immunostained for GM130 and Flag. Intensity plot corresponding to the region marked by a white arrow are shown on the right. Scale bar, 10 μm. Full size image The GM130–Cdc42 crosstalk involves RasGRF Another explanation for the GM130–Cdc42 connection could be that GM130 prevents the function of a Cdc42 inhibitor (schematic in Fig. 2 ). One possible candidate is the GEF RasGRF2, the RasGRF isoform expressed in epithelial cells, which has been recently shown to act as an inhibitor of Cdc42 (ref. 13 ). A marked association of endogenous GM130 and RasGRF2 could be detected in co-immunoprecipitation experiments ( Fig. 4a ). Moreover, in about 50% of the cells, RasGRF2 co-localized with GM130 at the juxtanuclear region, consistent with Golgi complex localization ( Fig. 4b,c ). RasGRF in addition also exhibited a localization pattern reminiscent of the ER, in agreement with previous work [24] . Noticeably, upon GM130 depletion, RasGRF2 juxtanuclear localization dropped strongly to <10% of the cells ( Fig. 4b,c ). Moreover we found that the interaction between these proteins was mediated by the C-terminal domain of GM130 and the Cdc25 domain of RasGRF2 ( Supplementary Fig. 6A,B ). These data suggested that GM130 is involved in localizing RasGRF to the Golgi complex. 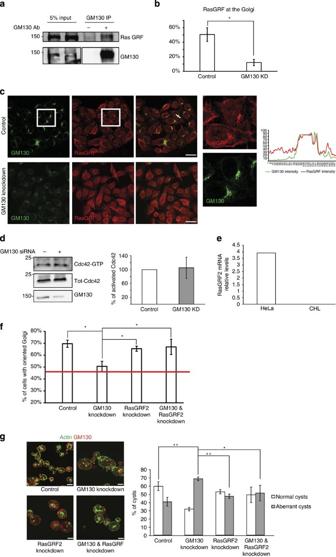Figure 4: The effect of GM130 on Cdc42 is dependent on RasGRF. (a) HeLa cells were lysed and the lysate was subjected to immunoprecipitation either with a GM130 antibody (+) or with protein G sepharose beads alone. ‘5% input’ indicates lanes where 5% of the total material that was used in the immunoprecipitation is loaded. (b) Quantification of cells with RasGRF at the Golgi. (c) Immunofluorescence staining in HeLa cells for RasGRF and GM130. Images were acquired using a confocal laser-scanning microscope. The magnifications correspond to the areas inside the white squares. Scale bar, 25 μm. An intensity plot corresponding to the region marked by a white arrow is shown. (d) CHL cells transfected with indicated siRNAs were lysed and GST-PAK1 was added to the lysate followed by pull down with GSH-sepharose. The eluate was subjected to immunoblotting against Cdc42 (Cdc42-GTP). Five per cent of the original lysate was immunoblotted against Cdc42 (Tot-Cdc42) and GM130. Bar graph represents a quantification of GTP-Cdc42 normalized to total Cdc42. Results are presented as mean±s.d. from three experiments. (e) Quantitative RT–PCR of RasGRF2 HeLa and CHL cells. (f) Confluent monolayer of cells transfected with the indicated siRNA was wound and cells were allowed to polarize for 6 h followed by fixation and staining of Giantin to label the Golgi. Golgis were counted as oriented towards the wound if their major mass was located in a 120° angle facing the wound. The red line shows the average orientation of the Golgi immediately after wounding. Results are presented as mean±s.d. from three experiments. (g) Caco-2 cells transfected with indicated siRNAs were grown in Matrigel for 4 days. Afterwards, cysts were stained for GM130 using immunofluorescence and for F-actin using phalloidin. Cysts with a single lumen were counted as normal, while cysts with multiple or no lumen were counted as aberrant. The percentage of normal and aberrant cysts in each condition was counted from three experiments which are displayed in the bar graph in the lower panel. Results are presented as mean±s.d. Scale bar, 7.5 μm. Statistics in F&G: analysis of variance with Newman–Keuls multiple comparison test (*P<0.05; **P<0.01). Figure 4: The effect of GM130 on Cdc42 is dependent on RasGRF. ( a ) HeLa cells were lysed and the lysate was subjected to immunoprecipitation either with a GM130 antibody (+) or with protein G sepharose beads alone. ‘5% input’ indicates lanes where 5% of the total material that was used in the immunoprecipitation is loaded. ( b ) Quantification of cells with RasGRF at the Golgi. ( c ) Immunofluorescence staining in HeLa cells for RasGRF and GM130. Images were acquired using a confocal laser-scanning microscope. The magnifications correspond to the areas inside the white squares. Scale bar, 25 μm. An intensity plot corresponding to the region marked by a white arrow is shown. ( d ) CHL cells transfected with indicated siRNAs were lysed and GST-PAK1 was added to the lysate followed by pull down with GSH-sepharose. The eluate was subjected to immunoblotting against Cdc42 (Cdc42-GTP). Five per cent of the original lysate was immunoblotted against Cdc42 (Tot-Cdc42) and GM130. Bar graph represents a quantification of GTP-Cdc42 normalized to total Cdc42. Results are presented as mean±s.d. from three experiments. ( e ) Quantitative RT–PCR of RasGRF2 HeLa and CHL cells. ( f ) Confluent monolayer of cells transfected with the indicated siRNA was wound and cells were allowed to polarize for 6 h followed by fixation and staining of Giantin to label the Golgi. Golgis were counted as oriented towards the wound if their major mass was located in a 120° angle facing the wound. The red line shows the average orientation of the Golgi immediately after wounding. Results are presented as mean±s.d. from three experiments. ( g ) Caco-2 cells transfected with indicated siRNAs were grown in Matrigel for 4 days. Afterwards, cysts were stained for GM130 using immunofluorescence and for F-actin using phalloidin. Cysts with a single lumen were counted as normal, while cysts with multiple or no lumen were counted as aberrant. The percentage of normal and aberrant cysts in each condition was counted from three experiments which are displayed in the bar graph in the lower panel. Results are presented as mean±s.d. Scale bar, 7.5 μm. Statistics in F&G: analysis of variance with Newman–Keuls multiple comparison test (* P <0.05; ** P <0.01). Full size image Overexpression of RasGRF1 or RasGRF2 blocked activation of Cdc42 at the Golgi as determined using the Cdc42-EM probe, in a manner dependent on the GEFs DH domain ( Supplementary Fig. 6C ). Importantly, co-knockdown of GM130 and RasGRF2 restored Cdc42 activation levels at the Golgi ( Fig. 1a ). The involvement of RasGRF in the GM130–Cdc42 crosstalk was further supported by the finding that GM130 depletion did not affect the levels of GTP-Cdc42 in CHL cells which naturally lack all RasGRF isoforms ( Fig. 4d ). Therefore, we conclude that RasGRF is an essential mediator in the GM130–Cdc42 crosstalk. Regulation of the GM130–RasGRF complex We hypothesized that GM130 could sequester RasGRF, thereby preventing it from binding and inhibiting Cdc42. Thus, under conditions that activate Cdc42, GM130 would sequester RasGRF to prevent it from inhibiting Cdc42. To test this hypothesis, we determined whether the GM130–RasGRF complex is affected by serum starvation, a condition under which Cdc42 is not activated. Under these conditions, GM130 did not co-immunoprecipitate with RasGRF ( Fig. 5a ), contrary to cells in steady state cultured under complete conditions ( Fig. 3 ). Treatment with 10% foetal calf serum (FCS) for 10 min resulted in re-formation of the GM130–RasGRF complex ( Fig. 5a ). If RasGRF were free under serum-starved conditions, then we would expect the Golgi pool of Cdc42 to be unresponsive to GM130 depletion. Cdc42 at the Golgi responded to serum treatment in control siRNA transfected cells, while GM130-depleted cells did not respond to this treatment ( Fig. 5b ). Of note, the FRET values at the Golgi were similar in control and GM130 silenced serum-starved cells, further supporting the notion that this pool becomes GM130-independent under serum-starved conditions ( Fig. 5b ). 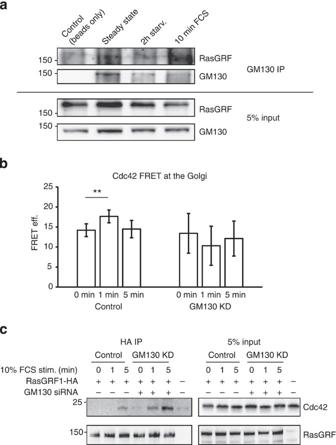Figure 5: The GM130–RasGRF complex is regulated by serum. (a) MCF7 cells were grown to confluency. Then, cells were serum starved for 2 h followed by stimulation with 10% FCS for the indicated time points. Cell lysates were subjected to immunoprecipitation against GM130. The immunoprecipitate was subjected to SDS–polyacrylamide gel electrophoresis followed by immunoblotting against the indicated proteins. (b) HeLa cells were transfected with control or GM130 siRNA 72 h prior to the experiment. After 48 h, cells were transfected with the plasmid encoding for the Cdc42 Raichu probe. Cells were serum starved for 2 h followed by stimulation with 10% FCS for 0, 1 and 5 min and FRET was measured as indicated in ‘Methods’. Results are presented as mean±s.d. from three independent experiments. Asterisks indicate statistically significant differences tested using analysis of variance with Newman–Keuls multiple comparison test (*P<0.05). (c) HeLa cells were transfected with the indicated siRNA. After 48 h, cells were transfected with empty vector or with a plasmid encoding haemagglutinin (HA)-tagged RasGRF1. After 24 h, cells were serum starved for 2 h followed by stimulation with 10% FCS for the indicated time points. Cell lysates were subjected to immunoprecipitation against HA. The immunoprecipitate was subjected to SDS–polyacrylamide gel electrophoresis followed by immunoblotting against the indicated proteins. Figure 5: The GM130–RasGRF complex is regulated by serum. ( a ) MCF7 cells were grown to confluency. Then, cells were serum starved for 2 h followed by stimulation with 10% FCS for the indicated time points. Cell lysates were subjected to immunoprecipitation against GM130. The immunoprecipitate was subjected to SDS–polyacrylamide gel electrophoresis followed by immunoblotting against the indicated proteins. ( b ) HeLa cells were transfected with control or GM130 siRNA 72 h prior to the experiment. After 48 h, cells were transfected with the plasmid encoding for the Cdc42 Raichu probe. Cells were serum starved for 2 h followed by stimulation with 10% FCS for 0, 1 and 5 min and FRET was measured as indicated in ‘Methods’. Results are presented as mean±s.d. from three independent experiments. Asterisks indicate statistically significant differences tested using analysis of variance with Newman–Keuls multiple comparison test (* P <0.05). ( c ) HeLa cells were transfected with the indicated siRNA. After 48 h, cells were transfected with empty vector or with a plasmid encoding haemagglutinin (HA)-tagged RasGRF1. After 24 h, cells were serum starved for 2 h followed by stimulation with 10% FCS for the indicated time points. Cell lysates were subjected to immunoprecipitation against HA. The immunoprecipitate was subjected to SDS–polyacrylamide gel electrophoresis followed by immunoblotting against the indicated proteins. Full size image If GM130 acts to protect Cdc42 from inhibition by RasGRF, then depletion of GM130 ought to increase the association between RasGRF and Cdc42. Co-immunoprecipitation experiments demonstrated that this was the case: the amount of RasGRF in association with Cdc42 increased in GM130 knockdown cells compared with control cells ( Fig. 5c ). Finally, we tested whether RasGRF is relevant for the GM130–Cdc42 crosstalk in the context of polarity. This was the case, as co-depletion of RasGRF2 and GM130 rescued the polarity defects imposed by GM130 depletion ( Fig. 3f,g ). The GM130–RasGRF complex controls Ras activity Our data indicate that GM130 acts as a repressor of RasGRF. Consistent with this model ( Fig. 6a ), knockdown of GM130 would release RasGRF, allowing it to inhibit Cdc42. However, RasGRF is also a well-known activator of Ras. Thus, loss of GM130 should also result in an increase of Ras activation. To test this prediction, we performed a knockdown of GM130 and measured Ras activation using a pull-down assay. Depletion of GM130 increased the levels of GTP-loaded Ras and co-knockdown of RasGRF abolished this effect ( Fig. 6b ), indicating that the increase in Ras activity was dependent on RasGRF. We also tested whether signalling downstream of Ras was modulated at the level of ERK1/2 in response to mitogen treatment. Knockdown of GM130 increased ERK1/2 activation in response to serum stimulation and this effect was again dependent on RasGRF ( Supplementary Fig. 7A ). To test whether the effect on ERK1/2 signalling is biologically relevant, we depleted GM130 in PC12 cells. These cells are a standard model for ERK-dependent cell fate decisions [25] . Higher and more sustained ERK1/2 signalling increases the likelihood that PC12 cells shift from proliferation to differentiation, which is evident by the emergence of neurites. Depletion of GM130 resulted in elevated and sustained ERK1/2 activation ( Supplementary Fig. 8A ) and accordingly the percentage of cells that underwent differentiation was significantly increased ( Supplementary Fig. 8B,C ). Thus, the effects of GM130 on Ras signalling are relevant for ERK-dependent cell fate decisions. 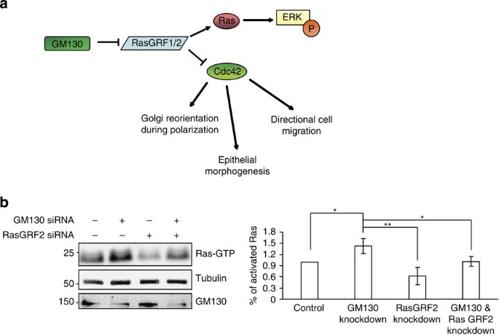Figure 6: GM130 depletion increases Ras activity. (a) Working model: GM130 acts as a suppressor of RasGRF activity, thereby modulating the activities of Ras and Cdc42. According to this model, the knockdown of GM130 results in increased Ras activation and decreased Cdc42 activation. (b) HepG2 cells were transfected with the indicated siRNAs. After 72 h, cells were lysed and Ras pull down was performed using GST-RBD. The eluate from the beads was subjected to SDS–polyacrylamide gel electrophoresis followed by immunoblotting with a pan-Ras antibody (Ras-GTP). Five per cent of the original lysate was subjected to SDS–polyacrylamide gel electrophoresis followed by immunoblotting against tubulin and GM130. Bar graph represents a quantification of the amount of active Ras (Ras-GTP) normalized to tubulin. Results are presented as mean±s.d. from three independent experiments. Asterisks indicate statistically significant differences tested using analysis of variance with Newman–Keuls multiple comparison test (*P<0.05; **P<0.01). Figure 6: GM130 depletion increases Ras activity. ( a ) Working model: GM130 acts as a suppressor of RasGRF activity, thereby modulating the activities of Ras and Cdc42. According to this model, the knockdown of GM130 results in increased Ras activation and decreased Cdc42 activation. ( b ) HepG2 cells were transfected with the indicated siRNAs. After 72 h, cells were lysed and Ras pull down was performed using GST-RBD. The eluate from the beads was subjected to SDS–polyacrylamide gel electrophoresis followed by immunoblotting with a pan-Ras antibody (Ras-GTP). Five per cent of the original lysate was subjected to SDS–polyacrylamide gel electrophoresis followed by immunoblotting against tubulin and GM130. Bar graph represents a quantification of the amount of active Ras (Ras-GTP) normalized to tubulin. Results are presented as mean±s.d. from three independent experiments. Asterisks indicate statistically significant differences tested using analysis of variance with Newman–Keuls multiple comparison test (* P <0.05; ** P <0.01). Full size image Expression of GM130 in colon cancer Loss of polarity is a frequent feature of epithelial tumours and is associated with dysplasia and increased metastatic potential [3] , [4] . Our results indicated that GM130 regulates polarity by modulating the Golgi pool of active Cdc42 and, in addition, Ras activity. Therefore, we asked whether GM130 might be associated with the malignant phenotype. To investigate this possible connection, we used two strategies. First, we analyzed GM130 expression in a colon cancer progression tissue microarray (TMA) comparing normal colon mucosa (29 cases), adenoma (16 cases) and adenocarcinoma (109 cases) ( Fig. 7a ). While the expression of GM130 only differed marginally in normal colon and adenoma, the expression in carcinoma was reduced markedly ( Fig. 7b–d ). We next extended this analysis to samples from 16 patients, present on TMA, with matched normal and cancer tissues. We compared the scored intensity of GM130 expression and found that in 14 out of 16 individual patients the expression of GM130 was reduced in tumours compared with the matched normal tissue ( Fig. 7e,f ). The downregulation of GM130 in cancer was further confirmed by an analysis of 11 matched normal and cancer colon tissues from a different source ( Supplementary Fig. 9 ). In this case, the intensity of the GM130 staining was measured and healthy tissues were compared with the matching cancerous tissues. In agreement with the previous results, GM130 was downregulated in the cancerous tissue in 9 out of 11 patients ( Supplementary Fig. 9A–C ). 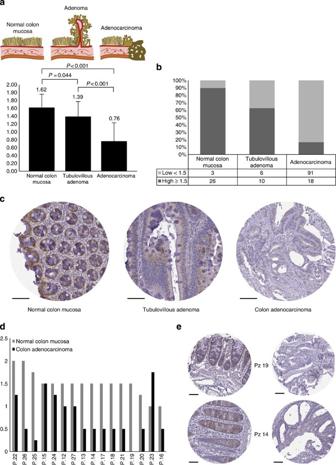Figure 7: Dysregulation of GM130 in human colon cancer. GM130 expression was measured by immunohistochemistry on a Colon Progression TMA. (a) Graphic representation of the neoplastic evolution of colon carcinoma from the normal colon mucosa through the adenoma. (b) Bar graphs depicting the average expression level (± s.d.) of GM130 in Normal Colon Mucosa, Colon Tubulovillous Adenomas and Colon Adenocarcinomas or (c) the percentage of low and high GM130-expressing samples when using a cutoff score value of 1.5 (differences are significant as assessed by Pearson’sχ2-analysisP<0.001). (d) Representative images of immunohistochemical staining for GM130. (e) Bar graphs depict the expression score of GM130 in 16 patients for which matched normal and tumour tissue were available on the TMAs. GM130 is downregulated in colon cancer with respect to the normal colon mucosa in 14 out of 16 patients. (f) Representative core images of normal and tumour tissues from patients 14 and 19. Scale bar, 100 μm. Figure 7: Dysregulation of GM130 in human colon cancer. GM130 expression was measured by immunohistochemistry on a Colon Progression TMA. ( a ) Graphic representation of the neoplastic evolution of colon carcinoma from the normal colon mucosa through the adenoma. ( b ) Bar graphs depicting the average expression level (± s.d.) of GM130 in Normal Colon Mucosa, Colon Tubulovillous Adenomas and Colon Adenocarcinomas or ( c ) the percentage of low and high GM130-expressing samples when using a cutoff score value of 1.5 (differences are significant as assessed by Pearson’s χ 2 -analysis P <0.001). ( d ) Representative images of immunohistochemical staining for GM130. ( e ) Bar graphs depict the expression score of GM130 in 16 patients for which matched normal and tumour tissue were available on the TMAs. GM130 is downregulated in colon cancer with respect to the normal colon mucosa in 14 out of 16 patients. ( f ) Representative core images of normal and tumour tissues from patients 14 and 19. Scale bar, 100 μm. Full size image In support of a role for GM130 loss in tumour progression, we found that knockdown of GM130 in Caco-2 cells led to a loss of E-cadherin expression ( Supplementary Fig. 9D ), a phenotype that is often considered to be linked to tumour progression and a loss of epithelial identity and is in line with the notion that loss of polarity is a typical phenomenon in epithelial–mesenchymal transition [26] . We could show that the effect of GM130 on E-Cadherin was not cell line specific, as the depletion of GM130 also caused loss of E-Cadherin in another epithelial cell line ( Supplementary Fig. 9D ). A large body of research on directional migration and cellular polarization has focused on dissecting signalling events that originate from and are regulated by proteins at the plasma membrane. However, comparatively little is known about how polarity is regulated by signalling from endomembrane compartments like the Golgi apparatus. This organelle was shown to orient towards the leading edge in directionally migrating cells [27] and disrupting Golgi structural integrity resulted in a block of directional motility [8] . Our aim was to explore the functional relevance of the Golgi localized pool of Cdc42 (ref. 5 ). Overall, our data establish for the first time a role for active Cdc42 at the Golgi in the control of cell polarity and that the complex formed by GM130 and RasGRF is critical to this process. Of note, depletion of GM130 did not disrupt Golgi integrity or membrane trafficking, in agreement with several previous publications [28] , [29] . Different findings by others [30] , [31] , [32] might be attributable to the use of different cell lines, different siRNA concentrations and transfection reagents. We interpret our data to mean that the Golgi supplies the leading edge of migrating cells with active Cdc42. An alternative explanation could be that the Golgi is supplying the leading edge with a GEF for Cdc42, and recent work has speculated about such a possibility [33] . However, such a model cannot explain our data showing that co-depletion of RasGRF2 and GM130 rescues Cdc42 activation and cell polarity, which strongly implies that the presence of active Cdc42 at the Golgi is important for polarization. Thus, we consider it more likely that active Cdc42 is delivered from the Golgi to the leading edge. The Golgi could provide a permissive environment for accumulating active Cdc42 by being free or poor in GTPase activating proteins (GAPs). In fact, no Rho family GAPs were have been found at the Golgi, except for small amounts of ARHGAP21 (ref. 34 ); Oliver Rocks, personal communication). Recent computational modelling approaches have analyzed the contribution of polarized trafficking to polarization of Cdc42 in yeast [35] , [36] , [37] . While trafficking appeared to be an important component, endocytic removal of Cdc42 from the leading edge, its lateral diffusion and ‘off’ kinetics from membranes were also found to be a key factor. This is in line with work showing that directional polarity is found to be dependent on Arf6 (ref. 33 ) a GTPase known to regulate endocytosis [38] . Altogether, our findings establish for the first time a connection between endomembrane Cdc42 activity and cell polarity and allow us to propose a role for this regulation in neoplasia. The GM130–RasGRF–Cdc42 axis appears as a potentially valuable new therapeutic target and future work will elucidate whether the loss of GM130 observed in tumours is associated with a change in the invasive or metastatic potential of cancer cells. Cell culture and transfection HeLa, HEK293, HepG2 and MCF7 cells were purchased from ATCC and were cultured in Dulbecco’s modified Eagles medium (DMEM) supplemented with 10% FCS and 100 U ml −1 penicillin/streptomycin. RPE-1 cells were grown in DMEM/F12 supplemented with 10% FCS and 100 U ml −1 penicillin/streptomycin. MDA-MB-231 were cultured in RPMI supplemented with 10% FCS and 100 U ml −1 penicillin/streptomycin. PC12 cells were cultured in RPMI supplemented with 10% human serum, 5% FCS and 100 U ml −1 penicillin/streptomycin. Caco-2 cells were cultured in minimal essential medium supplemented with 20% FCS and 100 U ml −1 penicillin/streptomycin. To generate stable cell lines, cells were transduced with lentiviruses (produced according to the protocols of Trono’s lab) and transduced cells were either selected with antibiotics or sorted via fluorescence-activated cell sorting. Transfection of siRNA was performed using HiPerFect (Qiagen) or Lipofectamine2000 (Invitrogen) according to the manufacturer’s instructions. The siRNAs used for the GEF screening were purchased from Thermo Fisher Scientific. Control siRNA was purchased from Thermo Fisher Scientific (ON_TARGETplus Control pool—Cat. Nr. D-001810-10-20). The siRNAs against GM130 were from Thermo Fisher Scientific (ON-TARGETplus smart pool—Cat. Nr. L-017282-00—indicated in the text as siRNA1) and from QIAGEN (SI04235147—indicated in the text as siRNA2—and SI00429191, indicated in the text as siRNA3). The siRNA against RasGRF2 was from Qiagen (SI04329941). The siRNA against TUBA was from QIAGEN (SI04220237—used in Fig. 1b ). Plasmid transfection was performed using Fugene6 (Promega) according to the manufacturer’s instructions. Cells were typically transfected 24 h prior to the experiment. PC12 cells were transfected with FugeneHD according to the manufacturer’s instructions. Plasmids Cdc42-GFP-wt (nr. 12599), Cdc42-GFP-TN (nr. 12601) and Cdc42-GFP-QL (nr. 12600) were from Addgene (Klaus Hahn’s Laboratory [6] ). RasGRF1-HA, RasGRF2-FLAG, RasGRF1-ΔPH-DH, RasGRF1ΔCdc25, RasGRF2-ΔDH and RasGRF2-ΔCdc25 were described previously [13] . myc-GM130-ΔN690 was cloned using pcDNA 3.1 myc-His as backbone pL-Venus-Cdc42 was cloned using a modified version of pLVTHM as backbone. RAICHU-Cdc42-EM and RAICHU-Cdc42-PM were kind gifts from Dr Michiyuki Matsuda (the Kyoto University, Japan). The RUSH-MannII–GFP expressing HeLa cells, as well as the VSVG–GFP–RUSH plasmid were a kind gift from Dr Franck Perez [39] . Temperature-sensitive VSVGts045–GFP was a kind gift from Dr Kai Simons. Flag tag ARHGEF9, 11 and 12 were a gift from Dr Oliver Rocks. Lentiviral packaging plasmids were bought from Addgene (psPAX2 nr. 12260, pMD2.G nr. 12259 and pLVTHM nr. 12247, from Didier Trono’s laboratory). GM130 GIPZ short hairpin RNA (shRNA) was bought from Thermo Scientific (Clone ID: V3LHS_313361). GM130 rat shRNAs (RSH050521 nr 1 to 4) and Control shRNAs (MSH029723-CH1) were bought from Genecopoeia. pmTurquoise2-Golgi was from Addgene (nr. 36205, ref. 40 ). Pull-down experiments To pull down. active Cdc42 cells were lysed in buffer (25 mM HEPES pH7.5, 150 mM Nacl, 1% Nonidet-P-40, 10 mM MgCl 2 ). Purified Glutathione S-transferase (GST)-tagged effector domain of PAK1 immobilized on GSH-sepharose beads was added to the lysate that was pre-cleared by centrifugation at 21,000 g for 5 min at 4 °C. After 1 h incubation at 4 °C, beads were washed twice followed by boiling in sample buffer to elute bound material. To precipitate active Ras, the same procedure was used with the exception the purified GST-tagged Raf1-RBD immobilized to GSH-sepharose beads were added to the lysate. ERK1/2 activation assays HeLa or HEK293 cells (250,000) were plated in 35 mm dishes and transfected with siRNA at the same time (HiPerFect from Qiagen). After 72 h, cells were serum starved for at least 2 h. Cells were subsequently stimulated with 10% FCS followed by lysis in ice cold MAPK buffer (150 mM NaCl, 20 mM Tris-HCl pH7.5, 1% Triton X-100) supplemented with protease and phosphatase inhibitors. The amount of phosphorylated ERK1/2 was determined by immunoblotting. PC12 differentiation PC12 cells were plated at low density on Collagen-coated coverslips. 24 h later, cells were transfected with plasmids encoding either control shRNA or GM130 shRNA. Cells were then serum starved overnight. Cells were then stimulated with 10% nerve growth factor (NGF) and 1% human serum for 48 h, then coverslips were stained and fixed. Cells with neurites as long as the body length were scored as ‘differentiated’. Due to the presence of GFP in the plasmid encoding for the shRNAs, we were able to count only cells effectively transfected. To measure P-ERK intensity, cells were stimulated as described above for 0, 30 or 90 min and then stained. Antibodies and immunofluorescent labels Rabbit monoclonal anti-Cdc42 (dilution 1:300—Cat. Nr. 2466), rabbit polyclonal ERK1/2 (dilution 1:1000—Cat. Nr. 4695) and rabbit polyclonal against phospho-ERK1/2 (dilution 1:1000—Cat. Nr. 9101) were purchased from Cell Signalling. Mouse monoclonal GTP-Cdc42 was purchased from NewEast Biosciences (dilution 1:50—Cat. Nr. 26905). To stain for GTP-Cdc42, Image-iT, FX Signal Enhancer from Invitrogen was used according to manufacturer’s instructions. Mouse monoclonal anti-GM130 antibody was from BD-Biosciences (immunofluorescence (IF) dilution 1:1000—westernblot (WB) dilution 1:250—Cat. Nr. 610823). Rabbit monoclonal anti-GM130 was from cell signalling (dilution 1:500—Cat. Nr. 12480). Rabbit monoclonal anti-RasGRF (WB dilution 1:200—IF dilution 1:50—Cat. Nr. Sc-863) and Mouse monoclonal E-Cadherin antibody (dilution 1:500—Cat. Nr. 21791) were purchased from Santa-Cruz. Rabbit polyclonal anti-Giantin antibody was from Covance (dilution 1:1000—Cat. Nr. PRB-114C). Monoclonal ANTI-FLAG M2-Peroxidase (horseradish peroxidase) was from Sigma (dilution 1:2000—Cat. Nr. A8592). Mouse monoclonal anti-HA 12CA5 antibody was from Roche (WB dilution 1:4000—IF dilution 1:500—Cat. Nr. 11583816001). Mouse monoclonal anti-γ-tubulin (dilution 1:1000—Cat. Nr. Ab11317), Rabbit polyclonal anti TGN46 (dilution 1:1000—Cat. Nr. Ab50595) were from Abcam, Mouse monoclonal anti-GFP (dilution 1:1000—Cat. Nr. 11814460001) was from Roche. AlexaFluor647 Phalloidin (Cat. Nr. A22287) and AlexaFluor488 concanavalin (Cat. Nr. C11252) and AlexaFluor647HPA (Cat. Nr. L32454) were from Invitrogen. For immunofluorescence staining, cells were grown on glass coverslips. To stain for RasGRF, cells were fixed on ice with 4% formaldehyde for 10 min followed by permeabilization with PBS containing 0.05% Triton X-100 for 3 min at room temperature (RT). To stain for β-COP, cells were fixed with methanol-acetone (50/50) for 2 min on ice. For all other stainings, cells were fixed with 4% paraformaldehyde for 15 min at RT followed by permeabilization with PBS containing 3% BSA and 0.2% Triton X-100. Microtubule nucleation assay RPE-1 cells were plated on coverslips and transfected with siRNAs using HIPerFect. After 72 h, 0.1 mM HEPES pH 7.35 was added to the cells and the cells were then transferred on ice for 40 min. Then cells were put back at RT and fixed after 0, 3 and 4 min at RT in fixation/permeabilization buffer (10 mM citric acid, 0.05% tween 20, pH 6.0, paraformaldehyde 2% in buffer CB, 0.025% glutaraldehyde, 0.2% Triton X-100). Immunostaining was then performed using antibodies against GM130, TGN46 and Tubulin. Caco-2 Cysts Caco-2 cells were plated in 35 mm dishes. Twenty-four hours later they were transfected with siRNAs using Lipofectamine 2000. After an additional 24 h, cells were trypsinized and an additional siRNA transfection using Lipofectamine 2000 was performed. Cells (6 × 10 4 ) were re-suspended in 60% DMEM+40% Matrigel (previously thawed overnight on ice). Hundred microlitres of this solution was plated into eight-well chambers (BD-biosciences), incubated at 37 °C for 30 min and, once solid, Matrigel was covered with 400 μl of DMEM. Media was changed every other day. On the 4th day, culture cysts were fixed with 300 μl of paraformaldehyde (4%) for 30 min at RT, washed with PBS, permeabilized with 0.5% Triton X-100 for 10 min and washed with PBS containing 7.5 mg ml −1 glycine. Non-specific staining was blocked with 300 μl of blocking buffer (7.7 mM NaN 3 , 0.1% BSA, 0.2% Triton X-100 and 0.05% tween20) and afterwards the eight-well chambers were incubated overnight with the primary antibodies diluted in PBS containing 3% BSA. On the next day, cells were washed with blocking buffer and secondary antibodies+fluorescent phalloidin were added for 2 h at RT. Cells were washed again with blocking buffer and the plastic support was removed. A glass coverslip was put on the top of the matrigel and the samples were imaged. Confocal microscopy image analysis and FRET Microscopy was performed on a LeicaSP5 confocal laser-scanning microscope equipped with a Ludin chamber. Most imaging was performed using the × 63 objective (1.4 NA). Images were converted into TIFF files and analyzed using ImageJ. FRET was performed using the donor recovery after acceptor photobleaching method using the FRET-AB wizard of the Leica software. Acceptor (yellow fluorescent protein) fluorescence was bleached at 100% laser intensity, assuring a minimal extent of bleaching by 75%. To analyze FRET at the Golgi, we chose a region in the juxtanuclear region where the reporter accumulated. To test whether we could recognize the Golgi correctly when looking at the reporter, we initially performed experiments where we co-localized the reporter with Golgi markers and found that we could always recognize the Golgi accurately. To measure FRET at the plasma membrane, we chose random regions at the plasma membrane of cells grown up to 80% confluency. Briefly, cells were divided into four regions (quadrants of a Cartesian Coordinates Plane) and FRET was measured every time in one different region (the first cell was measured in the first quadrant, the next cell in the second quadrant, and so on). The only limitation we imposed was to avoid regions overlapping with neighbour transfected cells. ImageJ was used to process the images. Briefly, the process ‘subtract background’ was used on every image. If needed to improve visibility, brightness and contrast of the images were corrected (linearly) using the ‘adjust’ menu of ImageJ. Images coming from the same experiment were all modified the same way to leave the information unaltered. Merged images were created with the appropriate function of ImageJ, after correcting the single channel images as described above. GEF screening FRET measurements at the Golgi were performed in HEK293 cells expressing the Cdc42-EM probe. We calculated the CI95 of GM130 knockdown versus control cells according to: Any value below the CI95 (red line in Fig. 2 ) was considered a hit. Our previous measurements of control and GM130 knockdown cells were used to quantitate the CI95 with the formula described above. Cells (30–45) were measured for each condition from two to three independent experiments. The rationale for measuring at least 30 cells was based on our calculation that 18 data points (that is, cells) are necessary to distinguish a population that differs from the control by 80% of the GM130 effect. FRET of directional migrating cells HeLa cells were plated on glass coverslips and transfected with siRNA (HIPerfect). After 48 h, cells were transfected with plasmids encoding Cdc42-EM or Cdc42-PM FRET probes (Fugene6). After 72 h, a wound was made using a 200 μl pipette tip and cells were allowed to migrate at 37 °C for 6 h. Then cells were either fixed or incubated for 1 h at 20 °C and subsequently fixed. To measure FRET, we selected the region of the cells directly facing the wound and named it ‘front’. For regions designated as ‘rear’ we chose regions from the side of the cell opposing the wound. Up to three different regions were measured in the ‘rear’ and averaged. We did not detect any dependency on where we measured as long as the plasma membrane was opposing the wound. We avoided measuring FRET in regions overlapping with neighbour transfected cells. Video acquisition of VSVG–GFP vesicles HeLa cells were plated on glass coverslips and transfected with siRNA (HIPerfect). After 48 h, cells were transfected with plasmids encoding for the VSVG–GFP–RUSH (Fugene6). After 72 h, a wound was made using a 200 μl pipette tip and cells were allowed to migrate at 37 °C for 4 h. Then imaging was started and biotin was added to release the VSVG construct from the ER. Images were acquired every 1.5 s. Golgi orientation, cell migration and aPKC recruitment assay For Golgi orientation assays, cells were plated on glass coverslips. After 72 h, a wound was made manually using a 200 μl pipette tip. Cells were stained with antibodies–anti γ-tubulin and anti-giantin–immediately after wounding and after 6 h. For assays measuring aPKC recruitment to the leading edge, cells were fixed 1 h after wounding. For migration assays, cells were transfected with siRNA, and trypsinized after 48 h and plated into Ibidi chambers placed on glass cover slips. This insert consists of two chambers separated by a 600 μm wall. Removal of the insert generates a wound with a defined width of 600 μm. Twelve-thousand cells were plated into each chamber. After 6 h, the IBiDi insert was removed and cells were allowed to migrate at 37 °C for 24 h. Then, cells were fixed and stained with concanavalin-alexa 488. Coimmunoprecipitations Cells (1 × 10 6 ) were plated in 10 cm 2 cell culture dishes. After 24 h, cells were transfected. After an additional 24 h, cells were lysed in immunoprecipitation buffer (20 mM HEPES pH 7.3, 200 mM KCl, 0.5% Triton X-100), then centrifuged for 15 min at 20’000 g . The supernatant was incubated with protein G sepharose beads coupled to the appropriate antibodies. For anti-HA immunoprecipitation commercial anti-HA beads (Sigma) were used. After 2 h of incubation at 4 °C, beads were recovered by centrifugation, washed and the bound material was eluted by boiling in sample buffer. RUSH assay to study ER–Golgi trafficking The RUSH assay was performed as described previously [39] . Briefly, 250,000 HeLa cells stably expressing RUSH-ManII–GFP were plated in 35 mm cell culture dishes and transfected with siRNA (using HiPerFect from Qiagen). After 72 h, cells were either fixed directly or were treated with 40 μM of biotin for 1 h followed by fixation in 4% paraformaldehyde at RT. Reverse transcription PCR (RT–PCR) Total RNA was isolated from cells by using the Qiagen RNeasy kit. Complementary DNA was prepared from 100 ng total RNA by using the high capacity cDNA reverse transcription kit (Applied Biosystems) following manufacturer’s instructions. Quantitative PCR was performed by using Fast SYBR green PCR MasterMix (Applied Biosystems). RT–PCR was run on 7900HT Fast RT–PCR system (Applied Biosystems). Expression of each gene was normalized to the expression of ubiquitin and β-2-microglobulin. Specific primers for RasGRF2 were described in Jacinto et al. [41] . Primers for TUBA, ARHGEF9, ARHGEF11 and ARHGEF12 were designed using PrimerExpress. Immunohistochemistry Three micrometre slides cut from three different TMA block containing a total of 229 different formalin-fixed, paraffin-embedded samples from colorectal cancers ( n =133), tubulovillous adenomas ( n =27) and normal colonic mucosa ( n =69) were used (duplicate cores for each samples). The project was approved by the ethical committee of the Instituto Europeo di Oncologia (IEO). Samples were rehydrated through xylene and graded alcohols. Antigen retrieval was accomplished using 1 mM EDTA, 0.05% tween. After peroxidase block with 3% H 2 O 2 for 5 min, and block with 2% goat serum in PBS for 1 h, samples were incubated with primary antibodies (Mouse monoclonal anti-GM130 antibody, BD-Biosciences) in a 1:50 dilution for 60 min at RT in 2% goat serum. Immunocomplexes were visualized by the EnVision+horseradish peroxidase Rabbit (DAKO, K4011), and acquired with the Aperio ScanScope system. Duplicate cores for every sample were evaluated and then the scores were averaged and considered as weak expression (average score 0.5–1), moderate expression (average score 1.5–2), strong expression (average score 2.5–3) or as negative if they scored 0. Immunohistochemistry data for GM130 expression were available only for 29 normal colonic mucosa, 16 tubulovillous adenoma and 109 colorectal cancer samples, since in some cases, individual cores detached from the slides during the manipulations. Eleven matched colon cancer samples were analyzed at the University of Regensburg according to the following procedure: two micrometre slides cut from a TMA block containing 60 different formalin-fixed, paraffin-embedded samples from colorectal cancers ( n =20) and matched normal tissues ( n =40) were used. Immunohistochemistry of GM130 was carried out in a BenchMark ULTRA (VENTANA) autostainer according to the manufacturer´s instructions. Briefly, retrieval was done using a citrate buffer (pH 6.0) for 44 min. The anti-GM130 antibody was used in a 1:100 dilution and incubated for 32 min. The slides were detected using the ULTRA View DAB detection kit (VENTANA). Negative controls without primary antibody were included in each experiment. Statistical analysis The data were analyzed using Student t -test, χ 2 -test or analysis of variance test for multiple comparison in GraphPad Prism. All IF images are representative of at least three independent experiments. Western blot and IF evaluations are averages of at least three independent experiments. For TMA analysis differences between experimental groups were examined for statistical significance using the nonparametric comparisons for each pair using Wilcoxon Method ( Fig. 7b ) or Pearson χ 2 -test ( Fig. 7c ). Where applicable, data are expressed as average±s.d. TMA data analysis was performed using JMP 10.0 statistical software (SAS Institute, Inc.). How to cite this article: Baschieri, F. et al. Spatial control of Cdc42 signalling by a GM130–RasGRF complex regulates polarity and tumorigenesis. Nat. Commun. 5:4839 doi: 10.1038/ncomms5839 (2014).